Hidden topological order and its correlation with glass-forming ability in metallic glasses Unlike the well-defined long-range periodic order that characterizes crystals, so far the inherent atomic packing mode in glassy solids remains mysterious. Based on molecular dynamics simulations, here we find medium-range atomic packing orders in metallic glasses, which are hidden in the diffraction data in terms of structure factors or pair correlation functions. The analysis of the hidden orders in various metallic glasses indicates that the glassy and crystalline solids share a nontrivial structural homology in short-to-medium range, and the hidden orders are formulated by inheriting partial crystalline orders during glass formation. As the number of chemical components increases, more hidden orders are often developed in a metallic glass and entangled topologically. We use this phenomenon to explain the geometric frustration in glass formation and the glass-forming ability of metallic alloys. The inherent atomic packing modes of glassy solids remain one of the most interesting and fundamental problems in condensed-matter physics and materials science [1] , [2] . Although significant progress has been made and provided insights into the atomic-level structure and short-to-medium-range order in glasses [3] , [4] , [5] , [6] , [7] , [8] , [9] , [10] , [11] , [12] , [13] , [14] , the way of leading to the medium-range order is still unclear [5] , [6] , [7] , [8] , [9] , [10] . Does a universal rule exist that nature follows to construct a glass structure as what has been discovered for crystals? Is there any connection between glassy and crystalline structures? If so, what does the connection look like and how is the connection related to the properties of glassy solids? In fact, the connection between glassy solids and crystalline counterparts has been paid much attention for long time [15] , [16] , [17] , [18] , [19] , [20] , [21] , [22] . Since 1950s it has been noticed [15] that substances with complex crystal structures like glycerol and the silicates can be very much supercooled and will form glasses, whereas those with simple crystal structures such as gold can only be supercooled a very few degrees, implying a close correlation between crystalline structures and glass-forming ability (GFA) of materials [17] . It has been also perceived that the structures of metallic glasses could contain partial crystalline orders, which give rise to a ‘confusion’ or ‘frustration’ and can be a structural basis for supercooling [16] , [17] , [18] , [19] , [20] , [21] , [22] . Despite the substantial understanding, it is still not clear what the physical origin of such correlations is, hampering further understanding of the nature of glasses and their properties. A glassy state is usually obtained by supercooling a liquid fast enough to avoid crystallization. The amorphous nature of glassy solids is experimentally ascertained by X-ray diffraction, transmission electron microscopy or selected area electron diffraction [14] . Almost all kinds of glassy solids exhibit similar mazelike selected area electron diffraction pattern without any local lattice fringes and broad diffraction maxima characteristic in X-ray diffraction data [14] . However, the glassy solids are inherently different in atomic-level structures, demonstrated by their different response behaviours under certain conditions, for example, the diverse annealing-precipitated crystalline-phases [23] , [24] , [25] , the distinct mechanical strength and ductility [26] , [27] , [28] , [29] , [30] , [31] , and the different thermal stability against crystallization [32] , [33] , [34] . Unfortunately, such a difference of inherent structures in glassy solids cannot be easily differentiated from a trivial analysis of the experimental diffraction data. However, the diffraction data such as structure factors or pair correlation functions (PCFs) are not as trivial as they look like. On the contrary, some studies have demonstrated that plenty of structural information is hidden behind the data of structure factors or PCFs, for example, a global packing containing both spherical-periodic order and local translational symmetry has been revealed by analysing PCFs of many metallic glasses [9] . A fractal nature of medium-range order in metallic glasses was also found by examining the relationship between the first peak position in structure factors and atomic molar volumes in many metallic glasses [7] . In fact, the oscillation in the structure factors or PCFs is an indication that a certain order does exist in amorphous solids [7] . Therefore, a more refined scrutiny of the diffraction data is desirable to get deeper insight into the glassy structural features and find a clue to unveil the nature of the structures in different glasses. In this paper, we systematically analyse the arrangement of peak positions in PCFs scaled by the first peak position for several glassy solids, including two pure metallic glassy Fe and Ni modelled by molecular dynamics (MD) simulations. Distinct hidden orders of atomic packing formula in medium range in these pure glassy solids are unveiled to be inherited from body-centred cubic (bcc) order in glassy Fe and face-centred cubic (fcc) order in glassy Ni, respectively, reflecting a nontrivial structural homology between glassy and crystalline solids from the perspective of spherical periodicity. By analysing the partial PCFs of three two-component metallic glasses of CuZr, NiAl and NiCu, which are similar but have distinct GFA, via MD simulations, very different hidden orders are observed in each individual systems and also inherited from fcc or bcc order, indicating that the hidden orders are more complex in multicomponent metallic glasses. The different hidden orders in a multicomponent metallic glass may be entangled topologically. More different hidden orders lead to more complex topological entanglement. Further analysis indicates that the formation of the hidden orders during cooling and their topological entanglement produce the geometric frustration against crystallization and are closely correlated with the GFA of metallic alloys. A map of hidden orders developed in metallic glasses during glass formation is finally constructed, which provides new insights into the structural properties and structure–property relationship in metallic glass-forming liquids and glasses. 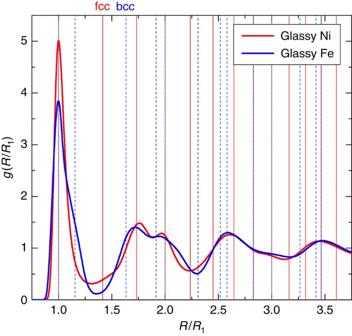Figure 1: MD modelled PCFs of glassy Ni and Fe at 300 K. The PCFs are scaled by the first peak positionR1. The characteristic constants in corresponding fcc and bcc crystalline lattice structures (denoted by solid and dashed vertical lines, respectively) are also presented. It shows a clear correspondence of the scaled peak positions in PCFs of glassy Ni and Fe with some characteristic constants of fcc and bcc lattice structures. Thus, a pure glassy solid may share the same ‘heart’ or similar atomic packing nature with its crystalline counterpart. Structural homology between monatomic glasses and their crystals Figure 1 shows the PCFs of glassy Ni and Fe at T =300 K scaled by the first peak position R 1 , respectively. It can be seen that at least five pronounced peaks are present in the range of about 1.2 nm, which indicates that there exists a structural order from short to medium range in glasses. We analysed the scaled peak positions R i / R 1 ( i =1,2,3,4,5) in PCFs by fitting each peak with a Gaussian function [9] . For glassy Ni, the values of R i / R 1 ( i =1,2,3,4,5) are 1.0, 1.74, 1.98, 2.64 and 3.46, respectively, quite close to the constants of , , , and . This is consistent with previous study [9] . We also carefully examined the values of R i / R 1 ( i =1,2,3,4,5) for glassy Fe and they are 1.0, 1.65, 2.0, 2.58 and 3.47, respectively. It is clear that the values of R 1 / R 1 , R 3 / R 1 and R 5 / R 1 are almost identical for glassy Ni and Fe, but the values of R 2 / R 1 and R 4 / R 1 are slightly different. We find that the values of R 2 / R 1 and R 4 / R 1 of glassy Fe are much closer to the constants of and , respectively, not and as in glassy Ni. All the data of the scaled PCFs in glassy Ni and Fe are summarized in Table 1 . Based on the above comparison, it can be concluded that the values of R i / R 1 ( i =1,2,3,4,5) in different glassy systems correspond to different constants. Now the questions are what these constants mean and what causes the difference. Figure 1: MD modelled PCFs of glassy Ni and Fe at 300 K. The PCFs are scaled by the first peak position R 1 . The characteristic constants in corresponding fcc and bcc crystalline lattice structures (denoted by solid and dashed vertical lines, respectively) are also presented. It shows a clear correspondence of the scaled peak positions in PCFs of glassy Ni and Fe with some characteristic constants of fcc and bcc lattice structures. Thus, a pure glassy solid may share the same ‘heart’ or similar atomic packing nature with its crystalline counterpart. Full size image Table 1 The first peak position R 1 and the relative atomic positions scaled by R 1 in the PCFs for glassy Ni and Fe obtained from MD simulations. 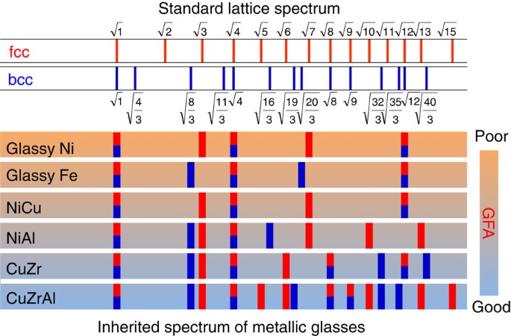Figure 2: The mapping of hidden orders in metallic glasses. The standard lattice spectra of fcc and bcc lattice structures are presented by short red and blue lines, respectively. Each line represents a characteristic constant in fcc or bcc lattice listed in the standard spectra and its position is determined accordingly. For metallic glasses, the scaled peak positions in the partial PCFs are the inherited characteristic constant sequence and marked with colour bars located at the positions of the corresponding characteristic constants. The colour of a bar is determined accordingly. The constructed map indicates that the hidden orders in metallic glasses are formulated by inheriting one or more characteristic constant sequences from the standard lattice spectra in crystalline structures. More characteristic constant sequences are often inherited in metallic glasses, as the number of chemical components increases, so that more different hidden orders are formed. The hidden orders in a metallic glass are closely correlated with the glass-forming ability of the metallic alloy. In the map, the metallic glasses investigated here are sorted with increasing the glass-forming ability (see Methods), which is illustrated schematically with the gradual colour change in the background. Full size table It has been demonstrated that the constants associated with the values of R i / R 1 ( i =2,3,4,5) in glassy Ni correspond to some relative atomic positions in fcc lattice structure [9] , so that we naturally examine the relative atomic positions of ( i =1–14) for fcc and bcc lattice structures, respectively, and the data are summarized in Table 2 . Here, ( i =1–14) denotes the distance of the i th nearest neighbour atoms. It is clearly seen that the values of ( i =1–14) are unique for fcc and bcc, respectively, and thereby reflect the characteristic atomic packing and structural feature of fcc and bcc lattice structures, so that they can be regarded as the characteristic constants in the corresponding lattice structures. Different lattice structures correspond to the different characteristic constant sequences. Table 2 Relative atomic positions scaled by the first peak position in four crystalline lattice structures. Full size table Comparing Tables 1 and 2 , it is found that the scaled PCF peak positions of R i / R 1 ( i =2,3,4,5) in glassy Ni correspond to some of the characteristic constants in fcc lattice structure, , , and . For glassy Fe, however, the constants associated the scaled peak positions in PCFs ( , , and ) belong to the characteristic constants in bcc lattice structure, not fcc. Figure 1 shows a clear correspondence of the scaled peak positions in PCFs of glassy Ni and Fe with some characteristic constants of fcc and bcc lattice structures, which are presented by solid and dotted vertical lines, respectively. Thus, it is clear that a pure glassy solid may share the same ‘heart’ or similar atomic packing nature with its crystalline counterpart. As only some characteristic constants in the crystalline counterparts are selected and associated with the scaled peak positions in PCF, a specific atomic packing order is formulated during glass formation and reserved in the glassy solid. Unlike crystalline counterparts, however, the specific atomic packing orders formulated in glasses are hidden in their broad distributions of PCFs or structure factors and cannot be directly detected in diffraction experiments. As PCF is an ensemble average of the distance distribution of atoms, the hidden orders are more related to the spherical-periodic order, but not orientational order. The nontrivial structural homology between one-component glassy solids and their crystalline counterparts inspired us to examine the hidden order in multicomponent metallic glasses. Hidden topological orders in multicomponent metallic glasses We did similar analysis for four model metallic glassy alloys of CuZr, NiAl, NiCu and CuZrAl by MD simulations, and the scaled peak positions of the partial PCFs in these systems were analysed. 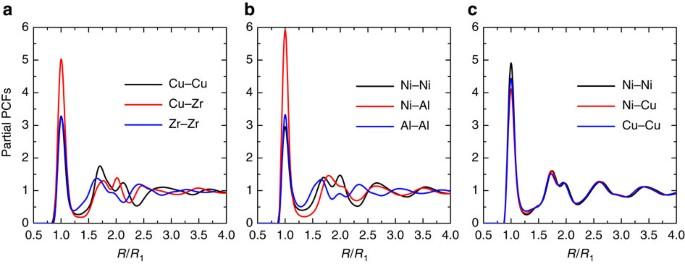Figure 3: The partial PCFs in three binary metallic glasses. The partial PCFs are scaled by the first peak positions. (a) In CuZr metallic glasses, the partial PCFs entangle with each other, implying that these hidden orders are entangled topologically. (c) In NiCu metallic glass, however, the scaled partial PCFs are almost collapsed together, indicating a very single hidden order, so that there is no order entanglement in this system. (b) The situation of NiAl metallic glass falls in between CuZr and NiCu. The results were summarized in Table 3 . As expected, the situation in multicomponent metallic glasses is much more complicated. For example, in CuZr metallic glass, the scaled peak positions of R i / R 1 ( i =2,3,4,5) in Cu–Zr partial PCF choose the characteristic constants of fcc lattice structure. The values of R i / R 1 ( i =2,3,4) in Cu–Cu partial PCF follow fcc order and choose the characteristic constants of fcc lattice structure, too, except the value of R 5 / R 1 (~3.67), which is much closer to a characteristic constant of bcc lattice structure, (see Table 2 ). Similar thing also occurs in Zr–Zr partial PCF, in which the values of R i / R 1 ( i =2,3,5) follow bcc order and choose the characteristic constants of bcc lattice structure, but the value of R 4 / R 1 (~2.41) is much closer to , which belongs to the characteristic constant sequence of fcc lattice, but not that of bcc lattice. Therefore, in Cu–Cu or Zr–Zr partial PCFs, the hidden order does not exactly follow fcc order or bcc order, but with fcc and bcc order hybridized. In addition, although the scaled peak positions of R i / R 1 ( i =2,3,4) in both Cu–Cu and Cu–Zr partial PCFs follow fcc order, R 4 / R 1 chooses different characteristic constants, in Cu–Cu and in Cu–Zr, which means that the hidden orders in Cu–Cu and Cu–Zr partial PCFs are different. Thus, three different hidden orders are identified in CuZr glasses. In NiAl metallic glass, the scaled peak positions of R i / R 1 ( i =2,3,4,5) in Ni–Ni and Ni–Al partial PCFs follow fcc order. Furthermore, they even choose the same characteristic constants of fcc lattice structure (see Table 3 ), which indicates that the hidden orders in Ni–Ni and Ni–Al partial PCFs are the same. For Al–Al partial PCF, the scaled peak position follow bcc order, different from Ni–Ni and Ni–Al. Therefore, we can conclude that there are two different hidden orders in NiAl glass. Note that in Al–Al partial PCF, the value of R 5 / R 1 (~3.11) is much closer to , which is the characteristic constant of fcc order, not that of bcc order. Therefore, a hybridization of fcc and bcc order also occurs in the hidden order in NiAl metallic glass. For NiCu metallic glass, surprisingly, the scaled peak positions of all partial PCFs follow fcc order, and even choose exactly the same characteristic constants of fcc lattice structure (see Table 3 ), which indicates that although NiCu metallic glass is two-component system, there exists a very simple hidden order, just like in one-component glassy solids. We also examine CuZrAl metallic glass, and a more complicated situation is expected, as a small amount of Al is introduced. As shown in Table 3 , the scaled peak positions of R i / R 1 ( i =2,3,4,5) in Zr–Cu, Cu–Cu and Cu–Al partial PCFs follow fcc order, but choose different characteristic constants of fcc lattice structure. This indicates that the hidden orders in Zr–Cu, Cu–Cu and Cu–Al partial PCFs are different. In Zr–Zr and Zr–Al partial PCFs, the scaled peak positions follow bcc order, but choose different characteristic constants, indicating two different hidden orders for Zr–Zr and Zr–Al atomic packing. Thus, there are total five different hidden orders in CuZrAl metallic glass. As shown in Table 3 , the value of R 4 / R 1 (~2.43) in Zr–Zr partial PCF is much closer to , which is the characteristic constant of fcc lattice, so that hybridization of fcc and bcc order exists in the atomic packing hidden order in Zr–Zr partial PCF. Table 3 The first peak position R 1 and the scaled peak positions by R 1 in partial PCFs of CuZr, NiAl, NiCu and CuZrAl metallic glasses obtained from MD simulations. Full size table Mapping of hidden orders in metallic glasses Based on the above analysis, it is clear that during glass formation, specific atomic packing orders are formulated in glassy solids according to the characteristic constant sequence of fcc or bcc lattice structures and hidden in the partial PCFs or diffraction data. Therefore, the characteristic constant sequences of fcc and bcc lattice structures can be designated as the standard lattice spectra. During glass formation, some of the characteristic constants are inherited from the standard lattice spectra, forming the specific atomic packing orders in glass structures hidden in diffraction data. Thus, a map of hidden orders in metallic glasses can be constructed as shown in Fig. 2 . The standard lattice spectra of fcc and bcc lattice structures are presented by short red and blue lines, respectively. Each line represents a characteristic constant in fcc or bcc lattice and its position is determined accordingly. For metallic glasses, the scaled peak positions in the partial PCFs are the inherited characteristic constant sequence and marked with colour bars located at the positions of the corresponding characteristic constants in the standard lattice spectra. The colour of a bar is determined accordingly. Thus, the map of hidden orders in metallic glasses is obtained. As shown in Fig. 2 , one-component metallic glasses inherit the fewest number of characteristic constants from the standard lattice spectra, and more and more characteristic constants are inherited in metallic glasses, as the number of component increases. For example, small addition of Al in CuZr leads to two more hidden orders and seven new characteristic constants inherited in CuZrAl metallic glass. Apparently different metallic glasses inherit different characteristic constant sequences. However, except the characteristic constant of , are inherited in all metallic glasses analysed here, so that it may be the most dominant structural element in metallic glass structures. in fcc lattice structure is another dominant one. On the other hand, some characteristic constants are never inherited in all metallic glasses, such as and in fcc and and in bcc lattice structures. Figure 2: The mapping of hidden orders in metallic glasses. The standard lattice spectra of fcc and bcc lattice structures are presented by short red and blue lines, respectively. Each line represents a characteristic constant in fcc or bcc lattice listed in the standard spectra and its position is determined accordingly. For metallic glasses, the scaled peak positions in the partial PCFs are the inherited characteristic constant sequence and marked with colour bars located at the positions of the corresponding characteristic constants. The colour of a bar is determined accordingly. The constructed map indicates that the hidden orders in metallic glasses are formulated by inheriting one or more characteristic constant sequences from the standard lattice spectra in crystalline structures. More characteristic constant sequences are often inherited in metallic glasses, as the number of chemical components increases, so that more different hidden orders are formed. The hidden orders in a metallic glass are closely correlated with the glass-forming ability of the metallic alloy. In the map, the metallic glasses investigated here are sorted with increasing the glass-forming ability (see Methods), which is illustrated schematically with the gradual colour change in the background. Full size image Note that in the standard lattice spectra, the characteristic constants from perfect hexagonal close-packed (hcp) lattice structure ( c / a = ) were not included. This is because most characteristic constants of perfect hcp lattice structure are included in those of both fcc and bcc lattice structures as shown in Table 2 . On the other hand, the characteristic constants in a specific hcp lattice structure depend on the ratio of c / a , which varies in different systems, so that they are not as generic as those in fcc and bcc lattice structures. Furthermore, we also examined diamond lattice structure and found that the characteristic constants in diamond lattice structure shown in Table 2 are all included in those of fcc and bcc lattice structures within the same relative distance, too. Therefore, the characteristic constants in fcc and bcc lattice structures are more fundamental and can be the representative of the standard lattice spectra. Now it is clear that for one-component glassy solids, only one characteristic constant sequence is inherited from their crystalline counterparts and forms the hidden order in these systems. For two-component glasses, more characteristic constant sequences could be inherited and thereby more hidden orders are formed depending on different systems. In CuZr glassy alloy, three different characteristic constant sequences are inherited and there are three different hidden orders. However, there are one and two characteristic constant sequences in NiCu and NiAl glassy alloys, respectively, forming different hidden orders. It is expected that more characteristic constant sequences are inherited and more hidden orders will be introduced as the number of chemical components of glassy alloys increases. Figure 3 shows the scaled partial PCFs in CuZr, NiAl and NiCu metallic glasses, respectively. In CuZr metallic glass, all three partial PCFs are distinct, which indicates the different medium-range atomic packing orders in Cu–Cu, Cu–Zr and Zr–Zr, respectively. As shown in Fig. 3a , these partial PCFs entangle with each other, implying that these hidden orders formed by the different characteristic constant sequences are entangled topologically in CuZr metallic glass. In NiCu metallic glass, however, the scaled partial PCFs are almost collapsed together as shown in Fig. 3c , indicating a very single hidden order, so that there is no order entanglement in this system. The situation of NiAl metallic glass falls in between CuZr and NiCu. The Ni–Ni and Ni–Al partial PCFs inherit same characteristic constant sequence and show similar pattern, but entangle with Al–Al one which inherits a different characteristic constant sequence. Therefore, if two or more characteristic constant sequences are inherited and different hidden orders are formed in glassy solids, the different hidden orders may lead to a topological entanglement, and more different hidden orders produce more complex topological entanglements. On the other hand, it can be seen that most characteristic constant sequences of hidden orders in metallic glasses are formed from either fcc or bcc standard lattice spectrum, as shown in Table 3 . In some characteristic constant sequences of hidden orders such as in Cu–Cu and Zr–Zr of CuZr glassy alloy, however, hybridization occurs, because they are combined with characteristic constants of both fcc and bcc lattice structures. Such hybridization in characteristic constant sequences of hidden orders in multicomponent glassy solids makes the hidden orders and the topological entanglement even more complicated. Figure 3: The partial PCFs in three binary metallic glasses. The partial PCFs are scaled by the first peak positions. ( a ) In CuZr metallic glasses, the partial PCFs entangle with each other, implying that these hidden orders are entangled topologically. ( c ) In NiCu metallic glass, however, the scaled partial PCFs are almost collapsed together, indicating a very single hidden order, so that there is no order entanglement in this system. ( b ) The situation of NiAl metallic glass falls in between CuZr and NiCu. Full size image The structural homology between glassy and crystalline solids and the topological entanglement of different hidden orders in glassy solids may be very important for understanding many critical aspects about nature of glass and glass transition, such as, the nature of atomic structures and medium-range atomic packing in metallic glasses and the GFA of metallic alloys. Because of the structural homology and the inheritance of hidden orders from standard lattice spectra, these critical issues in glassy solids could be pursued and understood from the crystalline view of point. It is commonly accepted that dense atomic packing promotes stability of the disordered phase and prevents crystallization of liquids. As demonstrated above, the structure homology of glassy solids may provide a new understanding of the atomic packing nature and medium-range order in metallic glasses. A recent study [35] also shows some interrelationships between the shear modulus of a metallic glass and that of the parent crystal, indicating their underlying structure similarity. On the other hand, the topological entanglement of hidden orders may be closely related to the GFA in glassy alloys. The topological entanglement of different hidden orders actually reflects a geometric frustration in medium range in glassy alloys. Complex entanglement indicates significant geometric frustration in medium-range atomic packing in glassy systems, which stabilizes the supercooled liquids against crystallization and leads to good GFA of metallic alloys. For example, significantly different GFA between CuZr and NiAl alloys has been found. The equivalent crystallization rates in these two alloys are remarkably different [32] . However, it is not arisen from some average properties of the bulk liquid structure and still far less understood [32] . In the picture of topological entanglement of different hidden orders, the significant difference in the GFA of CuZr and NiAl alloys can be well understood. During glass formation, more characteristic constant sequences are inherited and form more hidden orders in medium range in CuZr than in NiAl metallic glass. The different hidden orders are entangled together, so that the geometric frustration can be much more easily developed in CuZr alloy during glass formation. Thus, CuZr alloy has better GFA than NiAl. This picture can be confirmed in the case of NiCu. As shown in Table 3 , only a single characteristic constant sequence is inherited and one hidden order is developed in NiCu metallic glass during glass formation, and thereby no topological entanglement exists. Therefore, the geometric frustration cannot be developed in NiCu metallic glass during glass formation, resulting in very poor GFA in NiCu alloy. In our MD simulations, NiCu metallic glass can only be obtained by fast quenching with significant higher cooling rate compared with those used in ZrCu and NiAl alloys (see Methods). Therefore, more characteristic constant sequences are inherited to produce more hidden orders and complex order entanglement may lead to better GFA in metallic alloys. In experiments, minor alloying addition in metallic alloys is an effective way to increase GFA [36] , [37] , for example, the addition of small amount of Al in CuZr alloy can dramatically promote the GFA, and the experimental critical casting thickness increases from about 1 mm at composition of Cu 50 Zr 50 to about 8 mm at Cu 46 Zr 46 Al 8 (refs 37 , 38 ). According to the picture of the topological entanglement of hidden orders, more different hidden orders are introduced by adding Al atoms, which induces more characteristic constant sequences inherited from the standard lattice spectra, resulting in more complicated topological order entanglement, and thereby the geometric frustration, which significantly enhances the GFA in CuZrAl alloy. So far, to fabricate metallic glasses with good GFA, some empirical rules have been formulated, such as at least three components in alloys and significant atomic size difference among the constituent elements in alloys, the so-called confusion principles [39] . These empirical rules or the confusion principles are just practical implementation of the topological entanglement of different hidden orders, because more than three components can definitely introduce much more different hidden orders, which entangle together and more easily produce geometric frustration. In addition, it is much easier to introduce more hidden orders and realize a complex topological entanglement if the atomic sizes are significantly different among constituent elements. Thus, the different inherited characteristic constant sequences in hidden orders and their topological entanglement may be the structural origin of the empirical rules or the confusion principles for the fabrication of high GFA metallic alloys. Thus, the proposed map of hidden orders in metallic glasses and the picture of inheritance of characteristic constant sequences and order entanglement may provide a new understanding for systematically searching new alloys with good GFA in both experiments and computer simulations. In summary, we reveal a short-to-medium range atomic packing rule for metallic glasses by a systematic and refined scrutiny of the PCFs obtained from MD simulations. The results demonstrate that the atomic packing nature of glassy solids correlates tightly with the crystalline structures in the perspective of spherical periodicity, and structural homology exists between glassy solids and crystals. During glass formation, partial crystalline orders are inherited to formulate specific medium-range atomic packing orders hidden in the structure factors in glassy solids. Moreover, the development of the hidden orders in a metallic glass closely correlates with the GFA in metallic alloys by a topological entanglement of different hidden orders. This picture may provide a new perspective on the nature of glass and the structure–property relationship. However, there are still some critical issues need to be explored, for example, the composition-dependent hidden order in metallic glasses. How does the composition change the hidden orders and the order entanglement? To address these issues, more refined scrutiny of diffraction data is desired in future work. MD simulations In the MD simulations, the glass-forming process of two pure metals, Ni and Fe with fcc and bcc crystalline lattice structures, respectively, were investigated with embedded-atom method potentials [40] , [41] . The structure contains 10,000 atoms in a cubic box with periodic boundary conditions. In the glass-forming process, the sample was first melted and equilibrated at T =2,000 K for 2 ns (time step 2 fs) in NPT (constant number, pressure, temperature) ensemble, then cooled down to 300 K with a fast cooling rate (10 14 K s −1 ) to avoid crystallization, during which the box size was adjusted to give zero pressure. The temperature and pressure were controlled with Nose-Hoover thermostat and barostat, respectively. The cooled sample was further relaxed in NVT (constant number, volume, temperature) ensemble for 2 ns at 300 K and 1,000 configurations were extracted from the last 1 ns relaxation for structural analysis such as PCFs. Similar process was done for the systems of Cu 50 Zr 50 , Ni 50 Al 50 , Ni 50 Cu 50 and Cu 46 Zr 46 Al 8 alloys with recently developed embedded-atom method potentials [42] , [43] , [44] , [45] to generate glassy samples. All the simulations were performed using the LAMMPS package [46] . In the preparation process of metallic glass samples, the cooling rate of 10 12 K s −1 was used for CuZr, NiAl and CuZrAl liquids to get glassy states, which is much slower than that used to generate pure glassy Fe and Ni. For NiCu alloy, however, the cooling rate has to be as high as 10 13 K s −1 to generate glassy state of NiCu alloy in MD simulation. How to cite this article : Wu, Z. W. et al. Hidden topological order and its correlation with glass-forming ability in metallic glasses. Nat. Commun. 6:6035 doi: 10.1038/ncomms7035 (2015).